Systems-wide temporal proteomic profiling in glucose-starvedBacillus subtilis Functional genomics of the Gram-positive model organism Bacillus subtilis reveals valuable insights into basic concepts of cell physiology. In this study, we monitor temporal changes in the proteome, transcriptome and extracellular metabolome of B. subtilis caused by glucose starvation. For proteomic profiling, a combination of in vivo metabolic labelling and shotgun mass spectrometric analysis was carried out for five different proteomic subfractions (cytosolic, integral membrane, membrane, surface and extracellular proteome fraction), leading to the identification of ∼ 52% of the predicted proteome of B. subtilis . Quantitative proteomic and corresponding transcriptomic data were analysed with Voronoi treemaps linking functional classification and relative expression changes of gene products according to their fate in the stationary phase. The obtained data comprise the first comprehensive profiling of changes in the membrane subfraction and allow in-depth analysis of major physiological processes, including monitoring of protein degradation. For a complete understanding of physiological processes in a cell, the integration of tailored approaches addressing different levels of regulation is needed. Therefore Bacillus subtilis , a Gram-positive prokaryote serving as a model organism [1] , was subject to a wide range of transcriptomic [2] , [3] , proteomic [4] , [5] and metabolomic studies [6] , [7] . Unlike transcriptome analysis, proteomic studies do not necessarily cover all possible gene products of the cell. For a long time, the entirety of all proteins represented a far too complex mixture to be analysed at once, due to the large ranges of protein abundance, pI (isoelctric point), molecular weight, solubility or localization [8] . A recent example demonstrates that these limitations in analytics of large-scale proteomics can be overcome by application of different digest enzymes and gas-phase fractionation during mass spectrometry analysis [9] . Soluble proteins are the most intensively studied species of proteins due to their favourable accessibility. In two dimensional gel-based studies, the majority of the proteins localized in the cytosol, the extracellular space or the cell wall have been differentially accessed [10] . More effort has to be spent on proteins with multiple membrane-spanning domains, extreme pIs or molecular weights or with low abundance. In contrast to highly abundant soluble proteins [11] , [12] they need to be enriched and specifically analysed. Elaborate methodologies are known for subfractionation of cell extracts other than cytosolic proteins. Extracellular proteins secreted into the growth medium can be acid precipitated and subsequently analysed [13] . Cell wall bound and surface localized proteins are addressed by LiCl extraction and subsequent proteomic analysis via two dimensional gel electrophoresis [14] . Proteins from the cell surface of intact cells can be biotinylated and subsequently affinity purified [15] . Owing to the hydropathy and low abundance of the proteins [16] , the membrane proteome still represents one of the least accessible subproteomes. Proteomic analyses of membrane proteins of B. subtilis have been developed over a longer period of time [5] , [17] , [18] . Wolff et al. [19] and Hahne et al. [18] have proven that a combination of highly complementary enrichment and analytical techniques allows a very comprehensive analysis of the membrane proteome in Gram-positive bacteria. The aim of this study was the systems-wide profiling of compartment-specific changes on the proteome level in B. subtilis caused by glucose starvation. State-of-the-art complete metabolic labelling with stable nitrogen isotopes as described by MacCoss et al. [20] and high mass accuracy mass spectrometry were applied to retrieve a maximum level of proteomic data. We investigated cytosolic proteins, two different membrane fractions consisting of transmembrane and membrane-attached proteins (membrane-shaving fraction (MSF) and enriched membrane fraction (EMF)), proteins attached to the cell surface (biotinylation-enrichment fraction (BEF)) and secreted extracellular proteins (extracellular fraction) of B. subtilis . To substantiate and complement the proteomic profiling, transcriptome data were acquired together with the quantification of extracellular metabolites. The proteomic and transcriptomic data were visualized by using Voronoi treemaps to enable the intuitional accessibility and immediate comparison of the systems-wide data. In this study, we demonstrate temporal dynamic processes at the protein level that are so far unrivalled. Particularly, the temporal survey of membrane proteins in combination with the other more easily accessible subproteomes allows a broad monitoring of protein dynamics. The data reveal a comprehensive and unbiased overview on the physiological processes in B. subtilis as a model enabling in-depth analyses, including post-translational regulation of biosynthetic pathways, and an overview on time-dependent processes in the bacterial membrane as protein synthesis and degradation. Qualitative and quantitative analysis of the proteome Metabolically labelled B. subtilis proteins from growing and non-growing cells were fractionated to obtain five different subproteomes for a comprehensive view on regulatory and physiological changes ( Fig. 1 ). Entry into stationary phase was provoked by glucose deprivation at an optical density (500 nm) of 1 ( Supplementary Fig. S1 ). Based on our workflow, allowing highly accurate (average mass deviation of <2 p.p.m. in our analysis) and reliable data (0.11% false positives on average on protein level), we were able to considerably cover the proteome of B. subtilis . 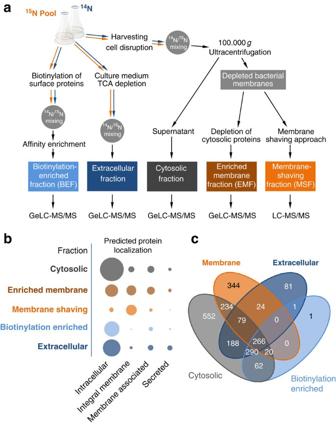Figure 1: Distribution of proteins identified according to the subfractionation workflow. (a) Workflow of the proteomic experiment. The preparation of the five different subcellular fractions is exemplified with the most crucial steps. The starting point for all proteomic samples is the bacterial batch cell culture. The first crossroads is the separation between complete cells for the BEF (biotinylation-enriched fraction) aiming at the surface-exposed proteins, the cell culture medium for the extracellular proteins and cells for the cytosolic/membrane fractions.14N/15N mixing depicts the stage in sample preparation, where mixing of the labelled pool and the unlabelled samples occurred. The earliest time point in experimental setup is chosen to minimize introduced effects by the labelling procedure to the quantitative data. Proteomic analyses (GeLC-MS and LC-MS) were performed with high-resolution and high mass accuracy mass spectrometry (2,142 total identified proteins with an FPR (false-positive rate) of 0.11% and 1.86 p.p.m. mass accuracy). (b) Distribution of proteins identified with a predicted subcellular localization in the different subfractions analysed. The area of the circles is proportional to number of identified proteins. (c) VENN plot of protein identifications in the different designated subcellular fractions. Numbers for the membrane fraction are summarized from EMF and MSF. Prediction of subcellular localization is according to Zhouet al.52Loci of localization assigned were as follows: intracellular; integral membrane proteins (multitransmembrane, multitransmembrane (lipid-modified N termini)); membrane-associated proteins (lipid anchored, LPxTG cell wall anchored, N-terminally anchored (no cleavage site), N-terminally anchored (with cleavage site), C-terminally anchored (with cleavage site), intracellular/TMH start after 60); secreted (secreted via minor pathways (bacteriocin) (no cleavage site), secretory (released) (with cleavage site)). In total, 2,142 proteins were identified with at least two peptides, which represents 52.2% of the entire predicted proteome ( Table 1 ; Supplementary Data 1 ). We were able to assign 552 proteins solely found in the cytosolic fraction ( Fig. 1 ), while 344 proteins were exclusively found to be associated with or completely inserted into the bacterial membrane. Furthermore, 81 proteins were identified only in the extracellular space. A substantial number of proteins were found in multiple subcellular fractions: 509 proteins were found in two, 389 in three and 266 proteins in all subproteomes. Figure 1: Distribution of proteins identified according to the subfractionation workflow. ( a ) Workflow of the proteomic experiment. The preparation of the five different subcellular fractions is exemplified with the most crucial steps. The starting point for all proteomic samples is the bacterial batch cell culture. The first crossroads is the separation between complete cells for the BEF (biotinylation-enriched fraction) aiming at the surface-exposed proteins, the cell culture medium for the extracellular proteins and cells for the cytosolic/membrane fractions. 14 N/ 15 N mixing depicts the stage in sample preparation, where mixing of the labelled pool and the unlabelled samples occurred. The earliest time point in experimental setup is chosen to minimize introduced effects by the labelling procedure to the quantitative data. Proteomic analyses (GeLC-MS and LC-MS) were performed with high-resolution and high mass accuracy mass spectrometry (2,142 total identified proteins with an FPR (false-positive rate) of 0.11% and 1.86 p.p.m. mass accuracy). ( b ) Distribution of proteins identified with a predicted subcellular localization in the different subfractions analysed. The area of the circles is proportional to number of identified proteins. ( c ) VENN plot of protein identifications in the different designated subcellular fractions. Numbers for the membrane fraction are summarized from EMF and MSF. Prediction of subcellular localization is according to Zhou et al. [52] Loci of localization assigned were as follows: intracellular; integral membrane proteins (multitransmembrane, multitransmembrane (lipid-modified N termini)); membrane-associated proteins (lipid anchored, LPxTG cell wall anchored, N-terminally anchored (no cleavage site), N-terminally anchored (with cleavage site), C-terminally anchored (with cleavage site), intracellular/TMH start after 60); secreted (secreted via minor pathways (bacteriocin) (no cleavage site), secretory (released) (with cleavage site)). Full size image Table 1 Proteins identified according to their predicted subcellular location. Full size table Subfractionation of the bacterial cell extract led to an enrichment of proteins with varying physical properties and different localizations. The proteins predicted as intracellular were found mainly in the cytosolic fraction ( Fig. 1 ). As expected, most integral membrane proteins were detected by using the membrane enrichment and the membrane-shaving approach. Membrane-associated proteins can be found primarily in the membrane-enrichment fraction and in the cytosolic fraction. The predicted secreted proteins could be identified to the highest extent in the extracellular fraction. Based on the identification data, we carried out a relative quantification with the software Census [21] . This software compares the 14 N mass traces of the respective samples with the 15 N mass traces of pooled labelled protein extracts used as a standard. Altogether, we were able to obtain quantitative data for 2,048 proteins. The quantitative results for every subfraction are provided in Supplementary Data S2 , S3 , S4 , S5 , S6 . Correlation of proteome and transcriptome data According to Becher et al. [22] three groups of proteins can be distinguished during the time course in cells entering the stationary phase: proteins no longer synthesized in non-growing cells but still present and relatively stable, proteins no longer synthesized and diminishing in amount, probably as a result of degradation, and proteins enriched in non-growing cells due to increased synthesis. In non-growing cells, many proteins are still present and probably (at least partially) active but no longer synthesized. The most significant advantage of a global proteomic study is that it yields information on the relative protein abundance, whereas transcriptomic studies monitor mRNA abundances as an indicator of changes in transcriptional activity and hence are unsuitable for capturing the protein inventory of cells. We combined both approaches and also performed an array-based transcriptome analysis under the same cultivation conditions to correlate our data on proteomic abundance with the corresponding transcriptional gene expression profiles. Visualization via Voronoi treemaps To support the analysis of our gene expression data from transcriptome and proteome levels, we used the functional gene categorization from KEGG orthology [23] , [24] and a structured representation of gene regulatory information derived from SubtiWiki [25] , [26] . Both schemes classify genes/proteins in an acyclic multihierarchical tree graph according to their function or regulation, respectively. For a well-arranged visualization, we adapted treemaps for an intuitive display of large omics data sets with their relative expression data and functional/regulatory classification ( Figs 2 , 3 ). 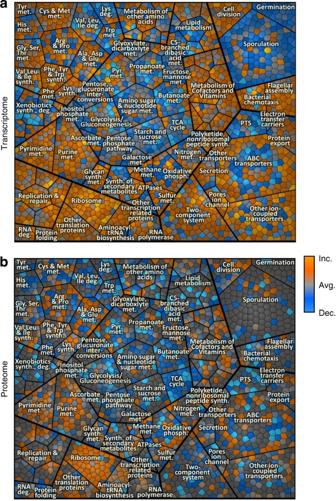Figure 2: KEGG-orthology treemap of growingB. subtilis. (a) Gene expression of growingB. subtiliscompared with average expression during the time course in cells entering the stationary phase. (b) Relative protein amount determined in cytosolic fraction of growingB. subtiliscompared with the average protein amount during the investigated time course. Each cell in the graph displays a single gene locus that belongs to other functionally related elements in parent convex-shaped categories. These are again summarized in higher-level categories. Functionally related elements seem in close neighbourhood to each other. Gene functional data are based on KEGG-orthology (for example, main level (metabolism)/first sublevel (carbohydrate metabolism)/second sublevel/(glycolysis)). To visualize differences in expression level/protein amount compared with the average level colour coding was applied as following: blue—decreased level (dec.), grey—same level as average (avg.), orange—increased level (inc.). These figures are part of the time course analysis (Supplementary Movies S1andS3), monitoring the changes from exponential growth to late stationary phase. Figure 2: KEGG-orthology treemap of growing B. subtilis . ( a ) Gene expression of growing B. subtilis compared with average expression during the time course in cells entering the stationary phase. ( b ) Relative protein amount determined in cytosolic fraction of growing B. subtilis compared with the average protein amount during the investigated time course. Each cell in the graph displays a single gene locus that belongs to other functionally related elements in parent convex-shaped categories. These are again summarized in higher-level categories. Functionally related elements seem in close neighbourhood to each other. Gene functional data are based on KEGG-orthology (for example, main level (metabolism)/first sublevel (carbohydrate metabolism)/second sublevel/(glycolysis)). To visualize differences in expression level/protein amount compared with the average level colour coding was applied as following: blue—decreased level (dec.), grey—same level as average (avg. ), orange—increased level (inc.). These figures are part of the time course analysis ( Supplementary Movies S1 and S3 ), monitoring the changes from exponential growth to late stationary phase. 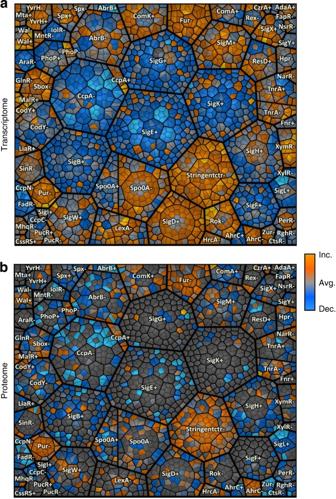Figure 3: Regulon treemap of growingB. subtilis. (a) Gene expression of growingB. subtiliscompared with average expression during the time course in cells entering the stationary phase. (b) Relative protein amount determined in cytosolic fraction of growingB. subtiliscompared with the average protein amount during the investigated time course. Each cell in the graph displays a single gene locus that belongs to other hierarchically/regulatory related elements in parent convex-shaped categories. These are again summarized in higher-level regulatory categories. Functionally related elements seem in close neighbourhood to each other. Treemap design is based on hierarchically structured regulatory data (black borders: regulon/thin black borders within the regulons: operon/smallest cells: gene). +/-; depict regulons being induced (+) or repressed (-;) depending on the regulator assigned to the area. To visualize differences in expression level/protein amount compared with the average level colour coding was applied as following: blue—decreased level (dec.), grey—same level as average (avg.), orange—increased level (inc.). These figures are part of the time course analysis (Supplementary Movies S2andS4), monitoring the changes from exponential growth to late stationary phase. Full size image Figure 3: Regulon treemap of growing B. subtilis . ( a ) Gene expression of growing B. subtilis compared with average expression during the time course in cells entering the stationary phase. ( b ) Relative protein amount determined in cytosolic fraction of growing B. subtilis compared with the average protein amount during the investigated time course. Each cell in the graph displays a single gene locus that belongs to other hierarchically/regulatory related elements in parent convex-shaped categories. These are again summarized in higher-level regulatory categories. Functionally related elements seem in close neighbourhood to each other. Treemap design is based on hierarchically structured regulatory data (black borders: regulon/thin black borders within the regulons: operon/smallest cells: gene). +/-; depict regulons being induced (+) or repressed (-;) depending on the regulator assigned to the area. To visualize differences in expression level/protein amount compared with the average level colour coding was applied as following: blue—decreased level (dec.), grey—same level as average (avg. ), orange—increased level (inc.). These figures are part of the time course analysis ( Supplementary Movies S2 and S4 ), monitoring the changes from exponential growth to late stationary phase. Full size image The treemap concept was established by Shneiderman [27] and originally served for the display of hierarchical structured data from software modules or file systems. His visualization is not based on a tree graph but on the planar combination of rectangular elements. Balzer and Deussen [28] improved this concept and developed Voronoi Treemaps, which use irregular, convex elements for treemap construction. This concept is very powerful and allows a visual perception of hierarchies that may contain several thousand elements. We adapted this concept [29] to link hierarchically structured regulatory (regulon/operon/gene) or gene functional data (for example, main level (metabolism)/first sublevel (carbohydrate metabolism/second sublevel/(glycolysis)) within Voronoi treemaps with data from gene expression measurements. Our treemaps combine areas representing functionally related elements in parent convex-shaped categories, which again become summarized in higher-level categories. After treemap construction and optimization, functionally related elements seem in close neighbourhood to each other. Expression data were visualized in the treemaps using a colour gradient: For illustration of protein expression level, colours of the range blue (lower than average) grey (equal to average) and orange (higher than average) were applied to Voronoi cells ( Figs 2 , 3 ). Most prominent examples of negative changes in protein amount belong to the nucleotide metabolism, the translational machinery and the biosynthesis of amino acids, as can be deduced from the Supplementary Movie S1 illustrating the proteomic cytosolic fraction. Proteins related to the degradation of amino acids and to the metabolism of carbohydrates increase in amount. The Supplementary Movie S2 displays the alteration of protein amounts with a treemap based on the transcriptional regulatory units. Regulons with many genes marking the cessation of exponential growth and the transition towards the stationary phase caused by glucose starvation are: the stringent control (consisting mostly of ribosomal proteins), PurR, Fur, FadR, SigL and CcpA. For a comparison and a comprehensive representation of processes taking place in the starving cell, the same visualization by Voronoi treemaps is provided for the transcriptome data in Supplementary Movies S3 and S4 . In-depth analysis of changes at proteome/transcriptome level In addition to the general overview on processes in the cell as provided by Voronoi treemaps, it is possible to monitor biological processes at the proteome level through in-depth analysis of the data. To follow the relative change in abundance throughout the complete time course for a specific protein, data for each protein were normalized to the first time point. The quantitative data were subjected to a significance analysis over the time course using analysis of variance. About a quarter of all identified proteins could be assigned to be significantly ( P -value<0.01) altered in amount ( Supplementary Data S2 , S3 , S4 , S5 , S6 ). As expected [7] , most obvious changes occurred for proteins of the carbohydrate metabolism: the key enzymes for gluconeogenesis, GapB and PckA, strongly increase in amount, whereas glycolytic enzymes of glycolysis remain relatively unaffected. Enzymes of the tricarboxylic acid cycle (TCA) increase more than twofold in protein amount ( Fig. 4 ). 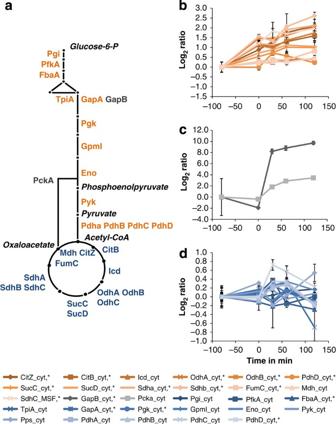Figure 4: Quantitative changes in proteins of the central carbon metabolism. (a) Graphical representation of the central carbon metabolism. The main metabolic intermediates are italicized. (b) Change of protein amount for glycolytic enzymes. (c) Change of protein amount for gluconeogenic key enzymes. (d) Change of protein amount for TCA enzymes. Error bars indicate s.d. of the biological replicates (n=3). Figure 4: Quantitative changes in proteins of the central carbon metabolism. ( a ) Graphical representation of the central carbon metabolism. The main metabolic intermediates are italicized. ( b ) Change of protein amount for glycolytic enzymes. ( c ) Change of protein amount for gluconeogenic key enzymes. ( d ) Change of protein amount for TCA enzymes. Error bars indicate s.d. of the biological replicates ( n =3). Full size image The proteomic profiles of several biosynthetic enzymes suggest that they undergo targeted degradation: besides the already known protease substrates [30] the data reveal PyrB, PurF, ArgG, ArgJ, LeuA, Sat and DhbC as new substrate candidates, according to the steeper slopes of decrease in protein amount compared with other members of functionally related biosynthetic pathways ( Fig. 5 ). The decrease in protein amount is in agreement with the decrease at the transcript level. 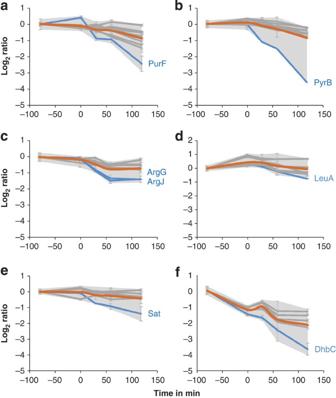Figure 5: Changes in proteins of the central carbon metabolism. Changes in protein amount for proteins of selected biosynthetic pathways. (a) Members of the purine biosynthetic pathway (PurR; PurB; PurK; PurN; PurH*; PurM;PurD*; PurL*; PurQ*; PurC*; PurF*). (b) Members of the pyrimidine biosynthetic pathway (PyrK; Pyre; PyrC*; PyrF;PyrAA*; PyrD; PyrAB; PyrB). (c) Members of the arginine biosynthetic pathway (ArgC; ArgD; ArgF*; ArgH*;ArgB; CarB; ArgG*; ArgJ*). (d) Members of the leucine/isoleucine biosynthetic pathway (LeuC; LeuD; IlvC; LeuB*;IlvB*; IlvH*; LeuA*). (e) Members of the cysteine biosynthetic pathway (YtiB; YvgQ; CysH; YvgR; CysC; Sat*). (f) Members of the bacillibactin biosynthetic pathway (DhbA*;DhbB*; DhbE*; DhbF*; DhbC*). Log2ratios are corrected for the first time point. Asterisks indicate proteins that are significantly altered as determined by analysis of variance (P-value<0.01). Error bars indicate s.d. of the biological replicates (n=3). Grey shading: area of maximal s.d. Orange: centroid of all proteins displayed. Blue: possible protease targets. Figure 5: Changes in proteins of the central carbon metabolism. Changes in protein amount for proteins of selected biosynthetic pathways. ( a ) Members of the purine biosynthetic pathway (PurR; PurB; PurK; PurN; PurH*; PurM;PurD*; PurL*; PurQ*; PurC*; PurF*). ( b ) Members of the pyrimidine biosynthetic pathway (PyrK; Pyre; PyrC*; PyrF;PyrAA*; PyrD; PyrAB; PyrB). ( c ) Members of the arginine biosynthetic pathway (ArgC; ArgD; ArgF*; ArgH*;ArgB; CarB; ArgG*; ArgJ*). ( d ) Members of the leucine/isoleucine biosynthetic pathway (LeuC; LeuD; IlvC; LeuB*;IlvB*; IlvH*; LeuA*). ( e ) Members of the cysteine biosynthetic pathway (YtiB; YvgQ; CysH; YvgR; CysC; Sat*). ( f ) Members of the bacillibactin biosynthetic pathway (DhbA*;DhbB*; DhbE*; DhbF*; DhbC*). Log 2 ratios are corrected for the first time point. Asterisks indicate proteins that are significantly altered as determined by analysis of variance ( P -value<0.01). Error bars indicate s.d. of the biological replicates ( n =3). Grey shading: area of maximal s.d. Orange: centroid of all proteins displayed. Blue: possible protease targets. Full size image The analysis of soluble proteins of the major metabolic pathways is well established and a wealth of information is known on B. subtilis coping with nutrient stresses. On the contrary, the membrane proteome covering the interface of the cell to the environment has been underrepresented in proteomic studies for a long time. For a broad understanding of processes in the model organism B. subtilis , this subgroup was included in the present study. Proteins involved in glycerol, ribose, lactate, nucleoside, succinate and fumarate uptake and zinc uptake exhibit an increased amount in the stationary phase. Conversely, a decrease was found for transporters of malate, Fe 3+ citrate, Fe 3+ hydroxamate, hydroxymethylthiamin (HMP)/thiamine transport and unknown substrates. ABC transporter systems found to be increasing in protein amount are specific for glutamate (GlnH/GlnQ), arginine (RocC, RocE) and for oligopeptides (YhjB, dpp and app operons). The major focus of this work is directed towards a global view on the processes on the proteome level in B. subtilis cells faced with glucose starvation. The combination of metabolic labelling with the existing toolbox of methods to access different proteomic subfractions opens up the possibility for systems-wide studies, previously only possible at the transcriptome level. Consequently, the analysis of 2,142 proteins regarding their dynamic change during a biological important process—the shift from growing to non-growing state—in a single study is a great step forward compared with previous studies of B. subtilis , such as Hahne et al. [31] , as reviewed by Wolff et al. [12] or as comprehensive studies most recently published by Soufi et al. [32] However, it has to be considered that gene products of lowly expressed genes are still underrepresented in our study ( Fig. 6 ). 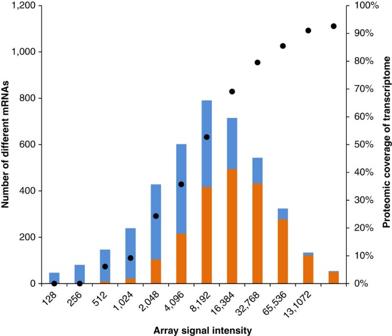Figure 6: Comparison of identified proteins depending on the maximum transcript intensities. The transcripts are binned according to their maximum array signal intensity over the whole time course. The number of genes belonging to the respective resembling group of transcript intensity is indicated in the bar chart in blue. Displayed in orange is the proportion of transcripts with accordingly identified translation products (proteins). The proteomic coverage of highly expressed genes is >90%, whereas for lowly expressed genes the coverage is significantly lower, as displayed with the circles on theyaxis on the right side. Figure 6: Comparison of identified proteins depending on the maximum transcript intensities. The transcripts are binned according to their maximum array signal intensity over the whole time course. The number of genes belonging to the respective resembling group of transcript intensity is indicated in the bar chart in blue. Displayed in orange is the proportion of transcripts with accordingly identified translation products (proteins). The proteomic coverage of highly expressed genes is >90%, whereas for lowly expressed genes the coverage is significantly lower, as displayed with the circles on the y axis on the right side. Full size image Despite our extensive fractionation scheme before mass spectrometric measurement, numerous proteins were additionally identified in other than the predicted subcellular fraction ( Table 1 ). For cytosolic proteins this can be explained by cell lysis after transition to the stationary phase and the still existing potential for improvement regarding the fractionation. In addition, overrepresentation of anticipated cytosolic proteins throughout the whole analysis may be explained by their increased analytical accessibility in our GeLC-MS (1D SDS Page coupled with LC-MS/MS analysis) approach and the high proportion of cytosolic proteins in the most abundantly transcribed groups. Furthermore, after imposition of starvation, cytosolic 'unemployed' proteins are prone to aggregation and degradation [30] , [33] . Proteins without substrates can form insoluble aggregates in the cell, which are spun down via ultracentrifugation after cell disruption in our preparation process, as was also observed by Hahne et al. [31] ( Supplementary Figs. S2-S4 ). In general, enrichment of proteins of a specific localization worked out well. Proteins belonging to a predicted subcellular location were found to the most extent in the corresponding subfraction of our workflow ( Fig. 1b ). A total of 1,511 cytosolic proteins were identified resulting in a considerable coverage of the 2,797 cytosolic proteins. The large set of quantitative data obtained for the cytosolic proteins enables a display with Voronoi treemaps, representing the main metabolic functional clusters in a single, intuitionally accessible graph. This avoids inherent shortfalls of shotgun proteomics yielding only tables with numerical values or representations; for example, by heatmaps lacking functional relatedness in visualization. Both orthology-based and regulon-based Voronoi treemaps consistently display changes on two complementary and physiologically meaningful levels of physiological regulation ( Figs 2 and 3 ). Necessary physiological regulation at the transition from exponential growth to the late stationary phase implies marked changes at the transcript and proteome level. Concomitant sampling of large-scale proteomics and transcriptomics data opens up the possibility for comparing both on a global scale. As expected, a correlation analysis of the two levels of regulation according to Fournier et al. [34] shows faster changes at the transcript level and a delayed cellular reaction on the proteome level ( Supplementary Fig. S5 ). The temporal offset of early mRNA and later protein changes could be related to the immediate cellular response on the transcript level and the time needed to accumulate the translated proteins. Accumulated proteins will then remain longer at their cellular localization contrary to their corresponding short-lived transcripts. The same situation holds true for mRNA/protein degradation: immediate responses towards decreased levels of mRNA are followed by slower degradation or even persistence of the protein species. The data obtained in this study reflect how glucose-starved cells modulate the metabolism by synthesis of new metabolic activity, degradation of specific components under starvation conditions and search for alternative nutrients. As a direct consequence of glucose depletion, the cells switch from glycolytic to gluconeogenic metabolism. This is based on the existing glycolytic pathway and additionally requires new enzymatic activity of glycerine aldehyde-3-phosphate-dehydrogenase (GapB) and phosphoenolpyruvate carboxykinase (PckA) [35] ( Fig. 4c ). Due to the importance of the TCA in stationary phase metabolism for energy generation, proteins of the TCA are induced significantly [7] . Regulation of expression of genes for the TCA in B. subtilis is complex [36] , [37] . Based on the proteomic data, regulation of the enzymes is in agreement with the knowledge so far [7] . Altogether, information about changes on proteome and transcriptome level for the main carbohydrate metabolism agree with already published data, underpinning the reliability of the data generated in the present work. Upon transition to the stationary phase, extensive reprogramming of gene expression takes place [3] , shutting down gene expression needed for exponential growth, including amino-acid biosynthesis, purine and pyrimidine synthesis and the translational machinery ( Supplementary Movie S3 ). Confirming the findings of Eymann et al. [38] and as displayed in Supplementary Movie S4 , genes of the stringent response are immediately downregulated by nutrient starvation. Ribosomal proteins as part of the negative stringent response regulon decrease markedly in protein amount ( Fig. 7 ), leading to a reduction <70% of the original amount of the ribosomal machinery inside the cell 2 h after nutrient depletion. The ribosomes contain a substantial fraction of intracellular protein content [39] , and consequently the degradation and recycling of amino acids represent a source of nutrients in times of starvation. 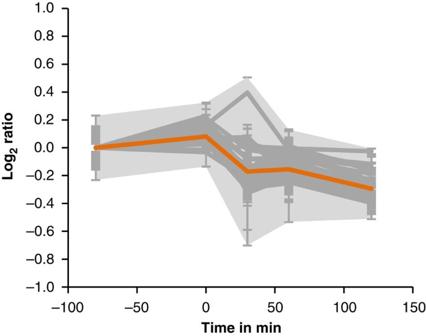Figure 7: Change of protein amount for ribosomal proteins from the cytosolic fraction. Relative quantitative changes for proteins belonging to the ribosome (YpfD; RpsL; RpsO; RpsJ*; RpmB; RpsP;*RpsD; RpsI; RpsH; RplD; RpsM*; RplB*; RpsE*; RpsF*; RpsR; RpsS; RpsG*; RpsT*; RplC*; RpmA; RplU*; RplR*; RplQ*; RpsQ*; RplE*; RplK; RpsB; RpmI; RplS*; RplF; RplI; RplX; RplW*; RpsK*; RplA*; RplP*; RplO*; RpsC; RplV*; RplT*; RplJ*; RplN*; RplL*; RplM*). Log2ratios are corrected for the first time point. Asterisks indicate proteins that are significantly altered as determined by analysis of variance (P-value<0.01). Error bars indicate s.d. of the biological replicates (n=3). Grey shading: area of maximal s.d.s. Orange: centroid of all proteins displayed. Figure 7: Change of protein amount for ribosomal proteins from the cytosolic fraction. Relative quantitative changes for proteins belonging to the ribosome (YpfD; RpsL; RpsO; RpsJ*; RpmB; RpsP;*RpsD; RpsI; RpsH; RplD; RpsM*; RplB*; RpsE*; RpsF*; RpsR; RpsS; RpsG*; RpsT*; RplC*; RpmA; RplU*; RplR*; RplQ*; RpsQ*; RplE*; RplK; RpsB; RpmI; RplS*; RplF; RplI; RplX; RplW*; RpsK*; RplA*; RplP*; RplO*; RpsC; RplV*; RplT*; RplJ*; RplN*; RplL*; RplM*). Log 2 ratios are corrected for the first time point. Asterisks indicate proteins that are significantly altered as determined by analysis of variance ( P -value<0.01). Error bars indicate s.d. of the biological replicates ( n =3). Grey shading: area of maximal s.d.s. Orange: centroid of all proteins displayed. Full size image As growth ceases, biosynthesis of amino acids is no longer needed. Besides the downregulation of biosynthetic genes, the protein amount of a large fraction of enzymes decreases. In concordance with transcriptomic data, enhanced degradation is seen for key enzymes of biosynthetic pathways. Noticeably, degradation rates for enzymes catalysing the first committed steps of biosynthetic pathways were higher than those of other constituents of the respective pathways ( Fig. 5 ). While such elevated protease-dependent degradation has been reported previously for PurF and PyrB [30] , our large-scale study adds new potential substrates for specific degradation (ArgG, ArgJ, LeuA, Sat and DhbC) that remain to be further investigated in future studies. The general stress response mediated by the alternative RNA polymerase sigma factor SigB provides the B. subtilis cell with multiple stress resistance strategies in anticipation of future stresses. The entire SigB regulon is induced directly after the transition to the starvation phase ( Supplementary Movie S4 ). Changes on transcript level for the sigB regulon are only reflected by six SigB-dependent general stress proteins on protein level. Besides the general stress marker proteins YvyD and GsiB, the proteases ClpC and ClpP increase in protein amount at the later time points 60 and 120 min after the transition. This is in good correlation with the increased protein aggregation and retrieval of aggregated cytosolic proteins in the EMF ( Supplementary Figs. S2-S4 ). Previous work revealed that a substantial number of membrane proteins is affected by amino-acid depletion or glucose downshift in the membrane of B. subtilis [40] . Indeed, we could detect major changes in the membrane proteome, so far only described in transcriptomic studies. Among the transporters that were diminished in protein amount, the major iron uptake systems revealed highly congruent changes (see Supplementary Fig. S6 ). The marked decrease imposed on the Fur [36] regulon suggests non-iron-limiting conditions. It remains to be elucidated if this is caused by the decreased biosynthetic activity of the cell compared with exponential growth. Remarkably, this notion is in accordance with data obtained for the closely related Staphylococcus aureus [22] . The largest group of induced transporter systems belongs to the CcpA regulon that is derepressed on cessation of growth due to the glucose downshift. The Supplementary Movies S2 and S4 of the regulon-based Voronoi treemap gives an impression of the complexity of derepression and/or substrate induction of CcpA-controlled operons and exemplifies changes of transporter proteins. Operons within the CcpA regulon are turned on in a sequential manner, resulting in a time-dependent insertion of new transporter proteins into the membrane (for details see Supplementary Figs S7-S14 ). Accordingly, most operons for catabolism of alternative carbon sources are under the transcriptional control of multiple layers of a regulating network that allows for fine-tuning by temporal dependence and strict order of preference. The high slopes of increase in protein amount result from the absence of most of the transporter proteins in the exponential growth phase. Taking the normalized spectral abundance factors (NSAFs) for these proteins into account, the final concentration of the respective proteins seems to be low in comparison with other transporters identified in the MSF (illustrated in Supplementary Fig. S15 ). It becomes clear that B. subtilis deploys new transport capacities for alternative carbon and energy sources at the onset of stationary phase, following glucose depletion to allow sensing and utilization of new nutrients. Interestingly, determination of extracellular metabolites reveals that most of the substrates of the newly installed transporter systems are absent or at least not detectable in our study ( Supplementary Fig. S1 ). A particular example is the induction of the citrate transporter CitM [41] . In contrast to the two other homologous uptake systems for different C4 TCA cycle intermediates, DctP [42] and MaeA [43] , no substrate is present in the medium during the entire cultivation and therefore substrate induction of CitM is not likely to take place. On the contrary, the malate transporter MaeA decreases in protein amount as a consequence of malate exhaustion in the growth medium. Furthermore, DctP increases markedly in amount in the stationary phase as its substrates, succinate and fumarate, accumulate in the medium during cultivation and are used as nutrients and building blocks in the starved cell. It remains to be elucidated if the substrates found in the growth medium cause antitermination/induction (degradation products of lysed bacteria or exported metabolites) or if an increase in protein amount is a consequence solely of derepression of the CcpA-mediated carbon catabolite repression. Similar to the temporal derepression of CcpA-dependent operons, parts of the Spo0A regulon were induced for a short time at the beginning of the stationary phase ( Supplementary Movie S3 ). Low-threshold induction of Spo0A genes leads to expression of the cannibalism operons skf and sdp ( Supplementary Fig. S16 ) [44] , [45] . The transient expression of genes and accumulation of these two systems—encoding among others, proteins being located at the cell membrane—to either protect the cell and to enhance/generate nutrient availability adds another important aspect of glucose starvation. Taken together, this work is the first global study that monitors time-dependent changes of integral membrane proteins of B. subtilis. Changes in the transport systems of the bacterial cell encountering limited nutrient availability are crucial switches for the adaptation of metabolic pathways and consequently for survival. Despite the short time of derepression/induction of the CcpA-regulated genes, it could be shown that new sets of nutrient uptake systems are inserted into the membrane. Preventive or substrate-induced provision of additional transporter specificity seems to be a major event after the onset of stationary phase following nutrient depletion in B. subtilis . To summarize, this work represents the first comprehensive study on concomitant transcriptome and large-scale proteome dynamics to be followed over five time points for B. subtilis coping with physiological perturbations. We monitored temporal and spatial changes at the proteome level covering all subcellular localizations in our global approach on glucose-starved B. subtilis to an unparalleled extent. So far, the analysis of soluble proteins of the major metabolic pathways has been well established and a wealth of information is known on B. subtilis coping with nutrient stresses. We were able to add qualitative and quantitative information gathered on the proteome level for the membrane proteome covering the interface of the cell to the environment that was underrepresented in proteomic studies for a long time. In this regard, time dependent insertion of additional substrate transporters into the membrane after glucose starvation could be shown. The combination of subfractionation techniques with state-of-the-art metabolic labelling and highly accurate mass spectrometry allows a more comprehensive overview of highly dynamic temporal and spatial processes in the model organism B. subtilis than was possible before. Most importantly, by concurrent sampling of large-scale proteomic and transcriptomic data, it was possible to reveal rapid alterations at the transcript level reflected at a slower rate of the proteome level, introducing new functionalities needed in stationary phase and degrading specific enzymes in biosynthetic pathways. Classification of proteins according to changes or stability was carried out and the implications for different physiological situations were shown. Elucidation of protein stability of specific pathways and the underlying mechanism seem to be one of the most promising topics to follow-up. It could be shown that degradative processes involve different subcellular locations that should be involved in future studies on targeted degradation in B. subtilis and its relatives. Systems-wide quantitative proteomic studies are valuable tools to display the actual situation of the "players of life", the proteins, in a biological sample. We assume that due to the experimental setup and the strain used, that is widely spread among the Bacillus community, this work with its spectral and raw data available in open repositories will be the base for future targeted approaches in the Bacillus community and beyond. Bacterial growth and metabolic labelling B. subtilis wild-type strain 168 ( trpC2 ) [46] was grown aerobically at 37 °C in a synthetic minimal medium [47] supplemented with either 15 N-ammonium sulphate/ 15 N- l -tryptophan (0.078 mM, 98 atom % excess, Cambridge Isotope Laboratories) or 14 N-ammonium sulphate and 14 N- l -tryptophan. Glucose and l -malate were added to a final concentration of 0.05% each to induce glucose starvation after growth to an OD 500 of 1.0. Cells were collected by centrifugation at different time points along the growth curve (exponential growth, transition phase, transition phase +30, +60 and +120 min). Relative quantification based on metabolic labelling of cell extracts was carried out as published by MacCoss et al. [20] 14 N-labelled cells were prepared in triplicate to obtain three biological replicates ( n =3). Preparation of mixed metabolically labelled cell extracts The washed cells were disrupted mechanically in a French press (Simaminco SLM) and the cell debris was removed via centrifugation (14 000 g at 4 °C for 20 min). Subsequently, the protein concentration of the unlabelled 14 N-samples and the pooled 15 N-samples was determined. The same protein amount of the 14 N-unlabelled and labelled 15 N-pooled protein extracts were mixed to obtain a metabolically labelled cell extract for further fractionation procedures. Fractionation of metabolically labelled cell extracts Membrane proteins were enriched according to the protocol published in Eymann et al. [5] , leaving out the extraction of proteins by n-dodecyl-β- d -maltoside treatment. In brief, sedimented cell membranes are subjected to subsequent ultracentrifugation/washing steps, including washing of the pellets with high-salt and carbonate buffer resulting in the EMF that is depleted of cytosolic proteins. The cytosolic fraction represents the supernatant after the first ultracentrifugation step in the membrane-enrichment protocol. The preparation of the integral membrane peptides is described by Wolff et al. [19] Briefly, the bacterial membrane is spun down via ultracentrifugation, subjected to a carbonate washing step and digested with Proteinase K in urea to deplete all soluble loops from the membrane. Transmembrane domains resting in the cell membrane are subsequently digested with Chymotrypsin in a buffer containing a detergent (RapiGest, Waters Corporation) suitable in mass spectrometry-based workflows, resulting in the MSF. Preparation of extracellular proteins To analyse the extracellular proteome, proteins in the cell medium were acid precipitated according to Antelmann et al. [48] In brief, proteins in the supernatant were precipitated on ice over night by adding 10% TCA to the supernatant that resulted from cell gathering. The precipitate was washed thoroughly with ethanol and the resulting protein pellet was dissolved in urea/thiurea. After determination of protein concentration and pooling of the 15 N-labelled extracellular proteins, equal protein amounts of the 14 N-samples and 15 N-pooled samples were mixed to obtain the metabolically labelled extracellular fractions. Preparation of biotinylation-enriched proteins samples The biotinylation approach and enrichment of surface proteins were performed following the protocol published by Hempel et al. [49] In brief, labelled ( 15 N) and unlabelled ( 14 N) cells were collected by centrifugation and subsequently biotinylated by Sulpho-NHS-SS-Biotin on ice. After quenching of the reaction and washing, cells were mixed before cell lysis to obtain the metabolically labelled extract after the following cell disruption. Biotinylated proteins were affinity purified with NeutrAvidin agarose. Elution of the purified and washed biotinlyated proteins was carried out by adding reductive SDS sample buffer. Sample preparation and proteomics measurement Preparation of protein fractions and explanation of the workflow leading to mass spectrometric results is described in more detail in the Supplementary Methods . In brief, samples that were analysed by the GeLC-MS workflow (EMF, cytosolic fraction, extracellular fraction, BEF) were fractionated by 1D SDS Gel electrophoresis followed by tryptic digestion, as described in Dreisbach et al. [40] The membrane-shaving (MSF) samples were prepared according to Wolff et al. [19] The tryptic-digested proteins were subjected to a reversed phase C18 column chromatography operated on a nanoACQUITY-UPLC (Waters Corporation). Peptides were first concentrated and desalted on a trapping column. Mass spectrometry (MS) and MS/MS data were acquired with an online coupled LTQ-Orbitrap mass spectrometer (Thermo Fisher). The digests resulting from the membrane-shaving fraction were subjected to reversed phase C18 column chromatography operated on a nanoACQUITY-UPLC (Waters Corporation) with a one column setup online coupled with an LTQ-Orbitrap mass spectrometer (Thermo Fisher). Subsequent to sample preparation, samples were subjected to LC-MS/MS analysis as described in Supplementary Methods . All mass spectrometry raw data are deposited into the PRIDE database with accession numbers of 11382-11458 ( http://www.ebi.ac.uk/pride/ ). Data analysis The *.dta files extracted from *.raw files using BioworksBrowser 3.3.1 SP1 (Thermo Fisher Scientific) with no charge state deconvolution and deisotoping performed on the data were searched with SEQUEST version v28 (rev.12) (Thermo Fisher Scientific) against a B. subtilis target-decoy protein sequence database (complete proteome set of B. subtilis extracted from UniprotKB release 12.7 (UniProt Consortium, Nucleic acids research 2007, 35, D193-197) with a set of common laboratory contaminants) compiled with BioworksBrowser. The searches were performed in two iterations: First, for the GeLC-MS analyses the following search parameters were used: enzyme type, trypsin (KR); peptide tolerance, 10 p.p.m. ; tolerance for fragment ions, 1 a.m.u. ; b- and y-ion series; variable modification, methionine (15.99 Da); a maximum of three modifications per peptide was allowed. For the membrane shaving approach, the following search parameters were applied: enzyme type, none; peptide tolerance, 10 p.p.m. ; tolerance for fragment ions, 1 a.m.u. ; b- and y-ion series; an oxidation of methionine (15.99 Da) and a carboxyamidomethylation (57.02 Da) of cysteine were considered as variable modifications with a maximum of three modifications per peptide. In the second iteration, the mass shift of all amino acids completely labelled with 15 N-nitrogen was taken into account in the search parameters. Resulting *.dta and *.out files were assembled and filtered using DTASelect (version 2.0.25) (parameters GeLC-MS: -y 2 -c 2 -C 4 --here --decoy Reverse_ -p 2 -t 2 -u --MC 2 -i 0.3 --fp 0.005; parameters membrane shaving: --nostats -1 1.9 -2 2.2 -3 3.3 -4 3.75 -i 0.299 -a false -p 1 -y 0 -d 0.1 -t 2 -u –here). The protein false-positive rate was calculated for each analysis according to Peng et al. [50] Data analysis relative quantification The workflow for relative quantification was carried out according to MacCoss et al. [20] The cured search results served as the base for the further analysis using the software Census [21] to obtain quantitative data of 14 N-peaks (sample) and 15 N-peaks (pooled reference [20] ). The software extracts the respective mass traces of the two isotopologues within a defined scan range centred around the fragment scan, leading to successful identification of the respective peptide. The ratio of the peak intensities is subsequently calculated for all overview scans contained in the chosen peak boundaries. Peptide ratios and combined protein ratios are finally exported ( R 2 -values >0.7 and only unique peptides; proteins failing to be relatively quantified were checked manually in the graphical user interface for on/off proteins). Proteins relatively quantified with at least two peptides were taken into account for the subsequent analysis. All quantification results of a complete GeLC-MS run were median centred and ratios were log 2 -transformed and averaged over the biological replicates. Time course data for each protein were adjusted to the first time point as reference point; proteins without quantitative information for the first time point were not taken into account for a detailed discussion. For a more detailed description on data analysis, including combination of quantification results, normalization and analysis of variance, see Supplementary Methods . Normalized spectral abundance factors To estimate the relative proportion of transporter proteins within the MSF, the NSAFs were calculated for these proteins according to Zybailov et al. [51] In Brief, the NSAF for a protein is the number of spectral counts ( SpC ; the total number of MS/MS spectra accounting for this specific protein) divided by the length L of the protein and divided by the sum of SpC/L for all proteins in the proteomic experiment. The NSAF is a measure for the relative portion of a protein in a proteomic analysis and proportional to the protein amount in the sample. Prediction of protein localization Predictions of protein localization in the cell were assigned according to the LocateP algorithm [52] Voronoi treemaps Algorithms for treemap calculations have been established in JAVA1.6 by using the corresponding Java Development Kit and have been formerly described in detail [29] Extracellular metabolite sampling and measurement by 1 H-NMR Detection and determination of concentrations for extracellular metabolites is described in detail in Supplementary Methods . Transcriptome analysis Generation of transcriptome data is described in detail in Supplementary methods . The complete data set is accessible through GEO Series accession no. GSE24058 . How to cite this article: Otto, A. et al. Systems-wide temporal proteomic profiling in glucose-starved Bacillus subtilis . Nat. Commun. 1:137 doi: 10.1038/ncomms1137 (2010).